Nanoparticles that deliver triplex-forming peptide nucleic acid molecules correct F508delCFTRin airway epithelium Cystic fibrosis (CF) is a lethal genetic disorder most commonly caused by the F508del mutation in the cystic fibrosis transmembrane conductance regulator ( CFTR ) gene. It is not readily amenable to gene therapy because of its systemic nature and challenges including in vivo gene delivery and transient gene expression. Here we use triplex-forming peptide nucleic acids and donor DNA in biodegradable polymer nanoparticles to correct F508del. We confirm modification with sequencing and a functional chloride efflux assay. In vitro correction of chloride efflux occurs in up to 25% of human cells. Deep-sequencing reveals negligible off-target effects in partially homologous sites. Intranasal delivery of nanoparticles in CF mice produces changes in the nasal epithelium potential difference assay, consistent with corrected CFTR function. Also, gene correction is detected in the nasal and lung tissue. This work represents facile genome engineering in vivo with oligonucleotides using a nanoparticle system to achieve clinically relevant levels of gene editing without off-target effects. Cystic fibrosis (CF) is an autosomal recessive, multisystem disease caused by defects in the cystic fibrosis transmembrane conductance regulator (CFTR), an ion channel that mediates chloride transport. Lack of CFTR function causes obstructive lung disease, intestinal obstruction syndromes, liver dysfunction, exocrine and endocrine pancreatic dysfunction, and infertility. Since the sequencing and cloning of the CFTR gene in 1989 (refs 1 , 2 , 3 ), numerous mutations resulting in CF have been identified [2] , [4] . The most common mutation in CF is a three base-pair deletion (F508del) on chromosome 7, which results in the loss of a phenylalanine residue, causing increased degradation of the CFTR protein before it can reach the cell surface. Although CF is one of the most rigorously characterized genetic diseases, current treatment of patients with CF focuses on symptomatic management rather than correction of the genetic defect. Some studies have demonstrated increased F508del activity with agents such as curcumin [5] , [6] or histone deacetylase inhibitors [7] ; VX-770 increases the activity of the CFTR protein in patients who have the less common G551D mutation. Gene therapy has remained unsuccessful in CF because of challenges including in vivo delivery to the lung and other organ systems. In recent years, there have been many advances in gene therapy for treatment of diseases involving the haematolymphoid system, where harvest and ex vivo manipulation of cells for autologous transplantation is possible: examples include the use of zinc-finger nucleases targeting CCR5 to produce HIV-1-resistant cells [8] , correction of the ABCD1 gene by lentiviral vectors [9] and correction of severe combined immunodeficient using retroviral gene transfer [10] . In contrast, harvest and autologous transplant is not a readily available option in CF because of the involvement of the lung and other internal organs. As one approach, the UK Cystic Fibrosis Gene Therapy Consortium is testing liposomes to deliver plasmids containing cDNA encoding CFTR to the lung. Other clinical trials have used viral vectors for delivery of the CFTR gene with limited success (reviewed here ref. 11 ), or CFTR expression plasmids that are compacted by polyethylene glycol-substituted lysine 30-mer peptides [12] . Delivery of plasmid DNA for gene addition without targeted insertion does not correct the endogenous gene and is not subject to normal CFTR gene regulation, while virus-mediated integration of the CFTR cDNA could introduce the risk of nonspecific integration into important genomic sites. New gene delivery vectors include a chimeric Ad5F35 vector that showed much higher efficiency than traditional Ad5 vectors [13] . Researchers have demonstrated that treatment with the microRNA miR-138 leads to improved synthesis of CFTR -F508del (ref. 14 ), and have also shown that lentiviruses can be used for gene transfer to porcine airways [15] . Other current gene and cell therapy strategies have been recently reviewed [16] . We reasoned that an attractive approach for CF gene therapy would be site-specific gene editing and correction of F508del. Unlike the delivery of plasmids containing CFTR , which would be transiently expressed, or nonspecific viral integration, site-specific gene editing would correct CFTR at its endogenous site, resulting in permanent gene modification under normal regulatory control. Current approaches for site-specific gene editing include short fragment homologous recombination using DNA fragments containing the correct CFTR sequence that can recombine with F508del CFTR genomic DNA, resulting in gene correction [17] , [18] , [19] , including introduction of the F508del mutation into normal mouse lung [18] . Zinc-finger nucleases (ZFNs [20] ) have recently been used to insert a CFTR transgene at the CCR5 locus [21] and for modification of F508del at levels <1% in vitro [22] . CRISPR/Cas-9 technology has been used to correct F508del in intestinal organoids from CF patients in culture [23] , but with high off-target effects (one out of 25 surveyed genes in a single analysed clone). In addition, the efficiency of gene modification was low: ∼ 0.3% of treated organoids (3–6/1,400) had the desired modification [23] . In vivo delivery is an important challenge, which was not attempted in this prior work with CRISPR/Cas9 or ZFNs. In our approach, we use triplex-forming peptide nucleic acids (PNAs). PNAs are synthetic oligonucleotide analogues, resistant to protease and nuclease degradation, that can induce DNA repair on sequence-specific triplex formation at targeted genomic sites [24] , [25] . Targeted genome engineering using this technique has historically been at low frequencies. Modification of PNA molecules with cell-penetrating peptides allowed for direct in vivo delivery in a supF reporter transgenic mouse, resulting in gene correction up to 0.06% in vivo. Our previous work has shown that triplex-forming PNAs and short donor DNA fragments can be used to edit the human β-globin gene [26] and the CCR5 gene [27] . Work by Schleifman et al. [27] has demonstrated that tail-clamp triplex-forming PNAs, containing an extended Watson–Crick strand invasion domain for the formation of PNA/DNA/PNA triplexes, have increased activity for gene modification. Nanoparticles are an attractive delivery tool [28] because of the numerous avenues for improving and fine-tuning delivery, including decoration with targeting ligands or cell-penetrating peptides [29] , use of surface modifiers to avoid uptake by phagocytes [30] and exploration of polymer compositions and formulations to create vehicles for effective clinical application [31] . Recently, we have developed biodegradable poly(lactic-co-glycolic) acid (PLGA) nanoparticles for PNA delivery. Using this approach, we were able to achieve increased in vitro modification of human haematopoietic stem cells (up to 0.9%) [32] . Application of these nanoparticles for modification of the human CCR5 gene resulted in in vivo gene modification of up to 0.5% in the spleen [33] . Our group also developed a new method for surface-modifying PLGA nanoparticles with cell-penetrating peptides [29] , and found that this class of nanoparticles could deliver PNA molecules for inhibition of microRNAs in a lymphoma model [34] . This surface-modification strategy was combined with a polymer blend strategy for enhanced delivery of plasmid DNA to primary human lung cells in vitro [35] and importantly in vivo to epithelial airway cells in mice [36] . Enhanced delivery of nanoparticles to the lung type I epithelium and macrophages was seen using this polymer blend. Here we use tail-clamp PNAs and donor DNA molecules delivered in polymer nanoparticles to correct the F508del CFTR mutation both in vitro in human bronchial epithelial (HBE) cells and in vivo in a CF murine model. By combining our recently developed tail-clamp PNA and surface-modified polymer blend nanoparticle technologies, we achieve in vitro and in vivo gene correction an order of magnitude higher than previously achieved. Design of triplex-forming PNA molecules targeting CFTR We designed a donor DNA molecule homologous to the targeted region containing the F508del sequence, and three tail-clamp PNA molecules that bind near this site at homopurine/homopyrimidine stretches ( Fig. 1a,b ; Supplementary Fig. 1 ). A gel shift binding assay was used to confirm binding of these PNA molecules to the desired targets—successful binding is indicated by presence of a DNA band more proximally on the gel as the bound triplex-forming PNA molecule slows down the transit of the complex ( Fig. 1c ; Supplementary Fig. 1 ). Several bands may be present because of different binding configurations, as previously described [37] . We also designed an Allele-Specific PCR (AS-PCR) assay to differentiate between the integrated donor sequence and the endogenous F508del sequence, using plasmids for optimization and validation of the allele specificity of the PCR reaction ( Supplementary Fig. 2 ). Primers specific to the donor DNA selectively amplified the plasmid containing the donor sequence, whereas primers specific to the F508del sequence only amplified the plasmid containing the F508del sequence. Importantly, spiking of the PCR reaction on genomic DNA with excess donor DNA or excess PNA did not lead to a false-positive PCR artefact. However, spiking of the PCR reaction with donor DNA and PNA at high doses did result in inhibition of the PCR reaction ( Supplementary Fig. 2d ), suggesting that our AS-PCR may not pick up all samples with corrected genomes. We also noted occasional amplification of the F508del sequence with donor primers, which would not lead to false-positives or -negatives when trying to detect the donor sequence. Because of these limitations, AS-PCR was only used as an initial screening tool to identify active molecules before moving to sequencing and functional studies. 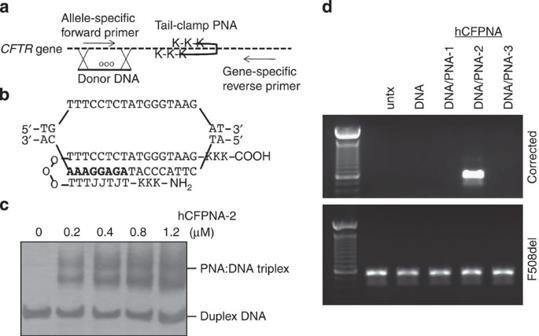Figure 1: Tail-clamp hCFPNA2 mediates correction of F508DEL in theCFTRgene. (a) Overall strategy for PNA-induced recombination and gene correction, and detection of modification by AS-PCR. (b) Schematic of hCFPNA2 forming a PNA/DNA/PNA triplex. J represents pseudoisocytosine, a C analog for improved triplex formation at physiologic pH. (c) Gel shift assay to test the binding of each designed PNA to the respective target site inCFTR: results for hCFPNA2. PNA was incubated with plasmid DNA with the targeted binding site, the binding region excised and the product analysed on PAGE gel with silver stain. (d) Human CFBE cells were treated with 2 mg ml−1nanoparticles for 24 h, and then harvested for genomic DNA extraction. AS-PCR was performed to detect the corrected sequence. Figure 1: Tail-clamp hCFPNA2 mediates correction of F508DEL in the CFTR gene. ( a ) Overall strategy for PNA-induced recombination and gene correction, and detection of modification by AS-PCR. ( b ) Schematic of hCFPNA2 forming a PNA/DNA/PNA triplex. J represents pseudoisocytosine, a C analog for improved triplex formation at physiologic pH. ( c ) Gel shift assay to test the binding of each designed PNA to the respective target site in CFTR : results for hCFPNA2. PNA was incubated with plasmid DNA with the targeted binding site, the binding region excised and the product analysed on PAGE gel with silver stain. ( d ) Human CFBE cells were treated with 2 mg ml −1 nanoparticles for 24 h, and then harvested for genomic DNA extraction. AS-PCR was performed to detect the corrected sequence. Full size image To screen PNA molecules for gene-editing activity, PLGA nanoparticles were loaded with PNAs and donor DNAs using a double emulsion solvent evaporation technique as previously described [32] . Nanoparticles with the donor DNAs alone, or DNAs and the various PNA molecules, were then tested on CF bronchial epithelial (CFBE) cells containing F508del (CFBE41o-) [38] . AS-PCR showed that F508del cells treated with PLGA nanoparticles containing both donor DNAs and hCFPNA2 had the desired modification present ( Fig. 1d ). Nanoparticles with donor DNA alone or with donor DNA plus either hCFPNA1 or hCFPNA3 were not effective. Confirmation of gene modification in isolated clones The nanoparticle-treated cell populations were seeded at limiting dilution into 96-well plates and expanded to isolate clones positive for the modification ( Supplementary Fig. 3 ). The frequency of modification in cells treated once with PLGA nanoparticles containing hCFPNA2 and the donor DNA, as calculated by limiting dilution analysis [39] , was 0.5–0.96%. Populations positive for CFTR gene correction were expanded by repeated limiting dilution to create more homogeneous clones, with the modification persisting over months of cell expansion. A 700-base-pair region around the modification site was amplified using PCR and sequenced, confirming the presence of the corrected sequence in clone 411 ( Fig. 2a ), and regular sequencing with limited PCR cycles revealed heterozygosity of the sample ( Supplementary Fig. 3c ), although with low sequencing quality. Higher-quality reads were obtained using deep-sequencing, which revealed that clone 411 was indeed heterozygous. Clone 411 was found to have 15897/35178 (45%) of alleles with the modified sequence, implying a heterozygous population with possibly a few contaminating unmodified cells (which may have remained even after the limiting dilution cell isolation process). 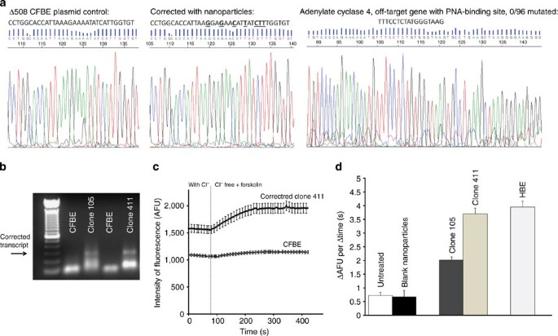Figure 2: Confirmation ofCFTRmodification in isolated clones. After human CFBE cells were treated with nanoparticles, modified clones were isolated by limiting dilution. (a) A 712-bp region around the modification site was amplified using PCR and sent for direct sequencing. A plasmid control with the uncorrected site, and cells corrected with nanoparticles (clone number 411 from limiting dilution cloning procedure) are shown. In addition, 96 clones of cells that were positive for the CF modification were analysed for off-target modification in the adenylate cyclase gene, which has partial homology to the PNA-binding site. No mutations were found. (b) Reverse transcriptase, allele-specific PCR using primers designed such that one binds to the corrected transcript and the other within the adjacent exon. The presence of a band indicates a transcript with the corrected sequence conferred by the donor DNA in corrected clone 411. Lower bands indicate nonspecific primer–dimer amplification. (c) The chloride efflux was measured using MQAE, a fluorescent indicator dye. Example traces from untreated CFBE41o- cells (n=23; bottom) and a corrected CFBE clone (n=26; top) are shown. Error bars, s.e.m. (d) Summary of the chloride efflux: cell-averaged AFU per min for untreated CFBE cells (n=138), blank-treated cells (n=168), modified clones (n=108 for clone 105,n=100 for clone 411) and wild-type 16HBE14o- cells (n=113). Error bars,s.e.m. Efflux rates of HBE cells (P<0.0001) and clone 105 (P=0.0061) and clone 411 (P<0.0001) were significantly different from that of untreated CF cells. There was no difference in the chloride efflux between untreated cells and those treated with blank particles. We used one-way analysis of variance with multiple comparisons to analyse the chloride efflux in untreated CF cells, blank particle-treated CF cells, clone 105, clone 411 and normal human bronchial epithelial cells (16HBE14o-). Figure 2: Confirmation of CFTR modification in isolated clones. After human CFBE cells were treated with nanoparticles, modified clones were isolated by limiting dilution. ( a ) A 712-bp region around the modification site was amplified using PCR and sent for direct sequencing. A plasmid control with the uncorrected site, and cells corrected with nanoparticles (clone number 411 from limiting dilution cloning procedure) are shown. In addition, 96 clones of cells that were positive for the CF modification were analysed for off-target modification in the adenylate cyclase gene, which has partial homology to the PNA-binding site. No mutations were found. ( b ) Reverse transcriptase, allele-specific PCR using primers designed such that one binds to the corrected transcript and the other within the adjacent exon. The presence of a band indicates a transcript with the corrected sequence conferred by the donor DNA in corrected clone 411. Lower bands indicate nonspecific primer–dimer amplification. ( c ) The chloride efflux was measured using MQAE, a fluorescent indicator dye. Example traces from untreated CFBE41o- cells ( n =23; bottom) and a corrected CFBE clone ( n =26; top) are shown. Error bars, s.e.m. ( d ) Summary of the chloride efflux: cell-averaged AFU per min for untreated CFBE cells ( n =138), blank-treated cells ( n =168), modified clones ( n =108 for clone 105, n =100 for clone 411) and wild-type 16HBE14o- cells ( n =113). Error bars,s.e.m. Efflux rates of HBE cells ( P <0.0001) and clone 105 ( P =0.0061) and clone 411 ( P <0.0001) were significantly different from that of untreated CF cells. There was no difference in the chloride efflux between untreated cells and those treated with blank particles. We used one-way analysis of variance with multiple comparisons to analyse the chloride efflux in untreated CF cells, blank particle-treated CF cells, clone 105, clone 411 and normal human bronchial epithelial cells (16HBE14o-). Full size image A region of an unrelated gene that has homology to the hCFPNA2-binding site, except for one-base-pair mismatch, adenylate cyclase type 4 on chromosome 14, was also sequenced, and no mutations were identified in 96 sequenced clones. While this regular sequencing in clones would not be able to identify mutations at a frequency lower than 1/96, additional experiments to ascertain off-target effects were performed in treated cells (see below). Correction of the CFTR gene was also confirmed using reverse transcriptase, allele-specific PCR on RNA extracted from a positive clone, as seen by the band corresponding to the modified sequence ( Fig. 2b ). Chloride efflux in the positive clones was quantified using N-[ethoxycarbonylmethyl]-6-methoxy-quinolinium bromide (MQAE), a fluorescent indicator dye, and perfusate solutions that switched from chloride-containing solutions to chloride-free solutions in the presence of forskolin and IBMX to maximally activate functional CFTR at the cell surface [40] , [41] . While untreated cells had minimal chloride efflux (flat line), the positive clones had increased chloride efflux in individually tested cells ( Fig. 2c ). The increased chloride efflux was calculated by measuring the rate of change in fluorescence over time (ΔAFU/Δs) as perfusate solutions were changed from chloride-containing to chloride-free solutions in the presence of a CFTR-stimulating cocktail. Chloride efflux was found to be significantly increased in the positive clones ( Fig. 2d ). Chloride efflux in clones was found to be similar to efflux in wild-type HBE cells, although there was some variations between clones. For instance, ‘clone’ 105, which had lower response, was found to have 350/8346168 of alleles modified in one deep-sequencing run, suggesting a heterogeneous population with variable expansion of modified cells. Improved in vitro activity of PLGA/PBAE/MPG nanoparticles Nanoparticles were then formulated from a blend of PLGA and 15% (wt%) poly (beta amino ester) (PBAE), surface-modified with the nuclear-localization sequence-containing cell-penetrating peptide MPG (modified PLGA/PBAE/MPG nanoparticles) [35] . Particles exhibited uniform size and morphology on scanning electron microscopy (SEM), and released most of their contents quickly, within the first 6–12 h of incubation in PBS at 37 °C, although there was more sustained release of nucleic acid cargo using the modified nanoparticles ( Supplementary Fig. 4 ). Increased uptake of fluorescently labelled PNA molecules was seen when PLGA/PBAE/MPG nanoparticles were used on human CFBE cells ( Fig. 3 ). 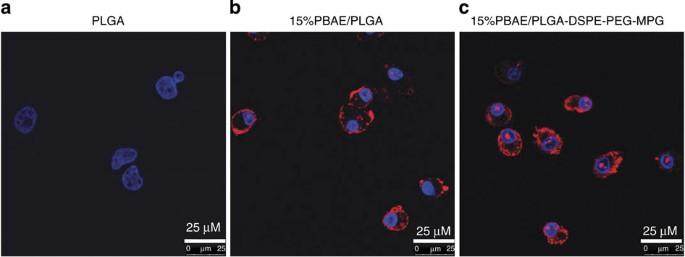Figure 3: Modified nanoparticles for increased PNA uptake. CFBE cells were plated on slides and treated with (a) 0.5 mg ml−1PLGA nanoparticles, (b) 0.5 mg ml−115% PBAE/PLGA nanoparticles or (c) 0.5 mg ml−115% PBAE/PLGA nanoparticles with MPG surface modification. All nanoparticles contained tamra-labelled PNA (red) and unlabelled DNA. Cells were stained with DAPI (blue) to track nuclear uptake. The Leica TCS SP5 confocal microscope was used to image cells. Figure 3: Modified nanoparticles for increased PNA uptake. CFBE cells were plated on slides and treated with ( a ) 0.5 mg ml −1 PLGA nanoparticles, ( b ) 0.5 mg ml −1 15% PBAE/PLGA nanoparticles or ( c ) 0.5 mg ml −1 15% PBAE/PLGA nanoparticles with MPG surface modification. All nanoparticles contained tamra-labelled PNA (red) and unlabelled DNA. Cells were stained with DAPI (blue) to track nuclear uptake. The Leica TCS SP5 confocal microscope was used to image cells. Full size image Change in chloride efflux was seen in CFBE cells serially treated three times with nanoparticles, without isolation of positive cells ( Fig. 4a ). Of note, interrogation of individual cells in these studies allowed us to quantify the absolute number of cells with functional chloride efflux. Approximately 7% of the PLGA-nanoparticle-treated cells demonstrated efflux similar to positive controls, and when CFBE cells were treated repeatedly with modified PLGA/PBAE/MPG nanoparticles 25% of cells demonstrated efflux equivalent to positive controls; this difference in modification efficiency was statistically significant ( P =0.003 two-tailed Fisher’s exact test). Cells treated similarly with PNA-carrying nanoparticles targeting a nonrelated genomic target or hCFPNA2 with a different donor DNA targeting a nonrelated genomic target did not have any change in chloride efflux ( Supplementary Fig. 5 ). Our previous work has suggested that this modified nanoparticle formulation is also optimal for in vivo delivery of cargo to the respiratory epithelium. We have recently shown that PLGA/PBAE/MPG nanoparticles are taken up by both macrophages and lung epithelial cells in mice [36] . 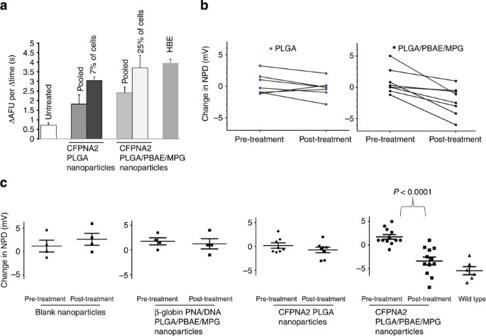Figure 4: Functional correction ofCFTRwith modified nanoparticlesin vitroandin vivo. (a) Summary of the chloride efflux: cell-averaged AFU per min for untreated CFBE cells (n=138), treated cells (n=150) and wild-type 16HBE14o- cells (n=113). F508del CFBE cells were plated at 10% confluence, and then treated three times with 2 mg ml−1particles over 7 days. They were then replated on slides and allowed 7–10 days to grow to confluence before the MQAE assay was performed to determine the chloride efflux. CFPNA2 NPs=cell population treated with PLGA nanoparticles containing hCFPNA2 and donor DNA. Seven percent of these cells exhibited efflux similar to positive HBE controls. CFPNA2-modified NPs=cell population treated with PLGA/PBAE/MPG nanoparticles containing hCFPNA2 and donor DNA. Twenty-five percent of these cells exhibited efflux similar to positive HBE controls.P=0.003 two-tailed Fisher’s exact test between PLGA and PBAE/PLGA/MPG-treated cells. Error bars show the s.d. (b) Mice were treated by intranasal infusion with nanoparticles. Nasal potential difference measurements were assessed before nanoparticle treatment, and subsequent to treatment. The response to a 0Cl+amiloride+forksolin perfusate after nanoparticle treatment was compared with the response before treatment. Each data point represents one mouse, with a line connecting pre- and post-treatment values. Mice treated with PLGA (left panel) or PLGA/PBAE/MPG nanoparticles (right panel) containing PNA/DNA are shown. Pre- and post-treatment changes in NPD were compared using pairedt-tests for each mouse. Treatment with PLGA nanoparticles demonstrated no difference in NPD; however, treatment with PLGA/PBAE/MPG nanoparticles demonstrated a significant change in NPD (P=0.004). (c) Nasal potential difference changes in functional and control nanoparticle treated CF mice. Each mouse is represented with an individual data point; in addition, the mean is shown with a horizontal line, surrounded by error bars showing the s.e.m. Pre- and post-treatment changes in NPD were compared using unpairedt-tests for each group. In the last panel, nasal potential difference changes in wild-type mice are shown for comparison. Figure 4: Functional correction of CFTR with modified nanoparticles in vitro and in vivo . ( a ) Summary of the chloride efflux: cell-averaged AFU per min for untreated CFBE cells ( n =138), treated cells ( n =150) and wild-type 16HBE14o- cells ( n =113). F508del CFBE cells were plated at 10% confluence, and then treated three times with 2 mg ml −1 particles over 7 days. They were then replated on slides and allowed 7–10 days to grow to confluence before the MQAE assay was performed to determine the chloride efflux. CFPNA2 NPs=cell population treated with PLGA nanoparticles containing hCFPNA2 and donor DNA. Seven percent of these cells exhibited efflux similar to positive HBE controls. CFPNA2-modified NPs=cell population treated with PLGA/PBAE/MPG nanoparticles containing hCFPNA2 and donor DNA. Twenty-five percent of these cells exhibited efflux similar to positive HBE controls. P =0.003 two-tailed Fisher’s exact test between PLGA and PBAE/PLGA/MPG-treated cells. Error bars show the s.d. ( b ) Mice were treated by intranasal infusion with nanoparticles. Nasal potential difference measurements were assessed before nanoparticle treatment, and subsequent to treatment. The response to a 0Cl+amiloride+forksolin perfusate after nanoparticle treatment was compared with the response before treatment. Each data point represents one mouse, with a line connecting pre- and post-treatment values. Mice treated with PLGA (left panel) or PLGA/PBAE/MPG nanoparticles (right panel) containing PNA/DNA are shown. Pre- and post-treatment changes in NPD were compared using paired t -tests for each mouse. Treatment with PLGA nanoparticles demonstrated no difference in NPD; however, treatment with PLGA/PBAE/MPG nanoparticles demonstrated a significant change in NPD ( P =0.004). ( c ) Nasal potential difference changes in functional and control nanoparticle treated CF mice. Each mouse is represented with an individual data point; in addition, the mean is shown with a horizontal line, surrounded by error bars showing the s.e.m. Pre- and post-treatment changes in NPD were compared using unpaired t -tests for each group. In the last panel, nasal potential difference changes in wild-type mice are shown for comparison. Full size image Correction of murine F508del in vivo To account for slight sequence variation between the mouse and human CFTR genes, new donor DNAs and PNAs were designed to target the mouse gene and correct the mouse F508del mutation. Binding of the mouse-specific PNA to the target DNA was confirmed using gel shift assay ( Supplementary Fig. 1 ). PLGA and PLGA/PBAE/MPG nanoparticles were formulated to contain the mouse-specific triplex-forming PNA and donor DNA, and CF mice [42] were treated with the nanoparticle suspension by intranasal application on days 1, 3, 6 and 9. Four days after the last treatment (day 14), correction of the mouse CFTR mutation in the nasal epithelium was assayed by measuring the nasal potential difference (NPD), a non-invasive assay used to detect chloride transport in vivo. Normally, CF nasal epithelia (human and mice) exhibit a large lumen-negative nasal potential that is amiloride-sensitive as well as a lack of activation of cyclic AMP-stimulated chloride efflux. This can be contrasted with a more modest amiloride-sensitive response and the presence of robust cyclic AMP-stimulated chloride efflux in non-affected tissue. The lack of activation of cyclic AMP-stimulated chloride flux is due directly to CFTR dysfunction and serves as a surrogate of CFTR activity. After intranasal delivery of mCFPNA2/donor DNA-containing nanoparticles, we found that the impaired response to cyclic AMP stimulation was partially corrected, with mice exhibiting NPDs that hyperpolarized in response to forskolin, which is more characteristic of wild-type mice ( Fig. 4b ). The degree of hyperpolarization in mice treated with unmodified PLGA nanoparticles containing mCFPNA2/donor DNA was modest and did not reach statistical significance. However, after intranasal delivery with PLGA/PBAE/MPG nanoparticles, we found that the response to cyclic AMP stimulation was much more robust, with mice exhibiting a significant increase in their response to forskolin ( Fig. 4c ). No significant change was seen in mice treated in parallel with blank nanoparticles, or in mice treated in parallel with PNA/DNA containing PLGA/PBAE/MPG nanoparticles targeting an unrelated genomic target but with similar base composition ( Fig. 4c ). In these control experiments, additional CF mice were treated identically to the experimental group with PLGA/PBAE/MPG nanoparticles containing either no nucleic acid cargo, or with PNA and DNA targeting human β-globin ; these PNA had similar base composition as the CF-targeted DNA but with 12 mismatches out of 17 in the Watson–Crick domain. The β-globin PNA was shown to be functionally active for inducing gene editing in β-globin [33] but had no effect on the CFTR gene. For comparison, cyclic AMP responses of the nasal potential difference assays in wild-type mice were more robust ( Fig. 4c ); this is expected given that wild-type mice have a homogenous population of wild-type CFTR -containing cells. In addition to the partial correction of the impaired cyclic AMP response, we observed a significant reduction in the large lumen-negative nasal potential in CF mice after treatment with PLGA/PBAE/MPG nanoparticles. This amiloride-sensitive portion of NPD was significantly reduced post treatment and similar in magnitude to that observed in wild-type mice ( Supplementary Fig. 6 ). Finally, there was no increased production of inflammatory cytokines in bronchoalveolar lavage (BAL) fluid of treated mice ( Fig. 5a ), and lungs showed normal histology ( Fig. 5b ). Histology of limited nasal epithelial samples showed no obvious differences between treated and untreated mice ( Supplementary Fig. 7 ). There was a reduction in inflammatory cells in the BAL of CF mice treated with PLGA/PBAE/MPG nanoparticles when compared with untreated CF mice: for n =4 mice in each group, average BAL cell counts were 1.24 × 10 5 in untreated CF mice, 0.4 × 10 5 in treated CF mice and 0.32 × 10 5 for wild-type mice, P =0.03 for untreated versus treated CF mice. 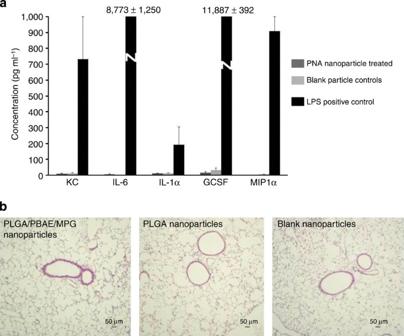Figure 5: Minimal inflammatory response with nanoparticle treatment. (a) Cytokine production in BAL fluid of treated and control mice, with BAL from lipopolysaccharide-treated control mice shown as a positive control, using Luminex bead-based assay. (b) Histology of treated and untreated mouse lungs, paraffin-embedded and stained with haematoxylin and eosin. Figure 5: Minimal inflammatory response with nanoparticle treatment. ( a ) Cytokine production in BAL fluid of treated and control mice, with BAL from lipopolysaccharide-treated control mice shown as a positive control, using Luminex bead-based assay. ( b ) Histology of treated and untreated mouse lungs, paraffin-embedded and stained with haematoxylin and eosin. Full size image Confirmation of modification with deep sequencing Modification was further confirmed in nanoparticle-treated human CFBE cells and in nanoparticle-treated mouse nasal epithelium and lung by deep sequencing, which allows for sequencing of millions of individual CFTR gene alleles in populations of cells ( Table 1 ). In human CFBE cells treated in vitro serially three times with PLGA/PBAE/MPG particles targeted modification frequency approached 10%. Increased efficiency of PLGA/PBAE/MPG nanoparticles over PLGA nanoparticles was also confirmed. In mice treated serially with PLGA/PBAE/MPG nanoparticles as described above, modification in the nasal epithelium was more than 5%, and more than 1% in the lung ( Table 1 ); modification was not detected in vivo when plain PLGA nanoparticles were used. In addition, deep sequencing of cDNA amplicons produced from lung mRNA detected at least greater than 80-fold higher expression of corrected CFTR RNA in a treated mouse (PLGA/PBAE/MPG particles) versus untreated, demonstrating that the modification was present at the mRNA level, consistent with our findings of functional correction. Table 1 Deep sequencing confirms efficient modification with low off-target effects. Full size table Off-target effects In addition, off-target modification in sites partially homologous to CFTR was examined. A section of chromosome 4 with 80% homology to the human donor DNA was queried in human cells (flanking features included a type II inositol-3,4-bisphosphate 4-phosphatase and a ubiquitin carboxyl-terminal hydrolase), and a similar section of the X chromosome with 50% homology to the donor DNA sequence (uncharacterized proteins) was queried in mice. In millions of sequenced alleles at these sites, there were no detected mutations above the machine-specific error rate ( Table 1 ). In addition, 13 additional off-target sites in the human genome with partial homology (>14 bp) to hCFPNA2 were queried in treated CFBE cells by deep sequencing. In these 13 additional sites, off-target mutation/error rates were similar to untreated controls ( Fig. 6 , Supplementary Table 1 ). For instance, for both untreated and treated cells, ∼ 80±15% (average across the 13 sites) of queried sequences had zero mismatches (no difference above the machine-specific error rate between samples), and similarly there were no differences in the number of sequences with one to five mismatches in the queried sites. No differences in mutation frequencies above the error rate were seen at the individual sites. Finally, a single-cell gel electrophoresis assay (comet assay) was used to assess for the presence of DNA double-stranded breaks ( Supplementary Fig. 8 ). In this assay, electrophoresis of lysed cells results in migration of fragmented DNA, producing images that resemble comets when observed using fluorescent microscopy, with the length of the comet ‘tail’ corresponding to the number of DNA breaks. No difference was seen between cells treated with DNA-containing and PNA/DNA-containing nanoparticles. In contrast, there was a slight but statistically significant increase in comet tail moments in cells treated with a human codon-optimized Cas9 expression plasmid [43] , which is designed to express CRISPR-associated protein 9, the DNA nuclease used in CRISPR-based gene-editing technologies that induces double-stranded breaks. 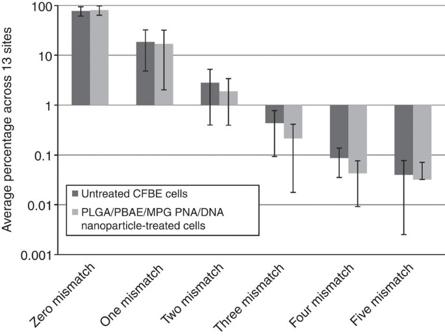Figure 6: Deep sequencing in additional human genomic sites showed no increased mutation rates in comparison with untreated controls. Two hundred-bp regions of DNA with partial homology to the PNA-binding site (>14 bps) in 13 disparate genomic sites were amplified using PCR, and PCR amplicons were sent for deep sequencing using the HiSeq (Illumina) 75-bp paired-end reads. CFBE cells treated three times with 2 mg ml−1PLGA/PBAE/MPG particles with PNA/DNA were compared with untreated CFBE cells. The total number of aligned sequences were queried, and the number of sequences with 0–5 mismatched based pairs. At each of the 13 off-target sites, the percentage of sequences that had 0–5 mismatched base pairs was calculated. The average and s.d. across the 13 genomic sites for 0–5 mismatches are shown. Mismatch percentages broken down by site are shown inSupplementary Table 1. Figure 6: Deep sequencing in additional human genomic sites showed no increased mutation rates in comparison with untreated controls. Two hundred-bp regions of DNA with partial homology to the PNA-binding site (>14 bps) in 13 disparate genomic sites were amplified using PCR, and PCR amplicons were sent for deep sequencing using the HiSeq (Illumina) 75-bp paired-end reads. CFBE cells treated three times with 2 mg ml −1 PLGA/PBAE/MPG particles with PNA/DNA were compared with untreated CFBE cells. The total number of aligned sequences were queried, and the number of sequences with 0–5 mismatched based pairs. At each of the 13 off-target sites, the percentage of sequences that had 0–5 mismatched base pairs was calculated. The average and s.d. across the 13 genomic sites for 0–5 mismatches are shown. Mismatch percentages broken down by site are shown in Supplementary Table 1 . Full size image We have developed a new approach for the treatment of CF, which combines novel PNA/DNA molecules targeting the common F508del mutation in CFTR both in vitro in HBE cells and in vivo in a CF mouse, with enhanced gene correction using modified nanoparticles. Three PNA molecules were designed to bind to the human CFTR gene at sites within 350 base pairs of the F508del mutation. These sites were chosen because homopurine/homopyrimidine sites are required for Hoogsteen binding and triple helix formation, and previous studies indicate that triplex-forming PNAs can increase levels of gene recombination at sites up to 750 base pairs (bp) from the target, with drop-off when the target is further than 400 bp away [44] . While all three PNA molecules we designed were found to bind to their respective targeted sites in CFTR , only hCFPNA2 was able to induce consistent gene modification in CFTR in conjunction with the donor DNA as detected using AS-PCR. In prior work, we have also noticed some variabilities in the ability of certain triplex-forming PNA molecules to induce gene modification [26] , [44] . Factors that may contribute to differences in PNA intracellular activity include accessibility of the binding site in the cellular chromatin, folding dynamics of the molecules being used, and strength of binding in intracellular conditions. Cloning by limiting dilution of nanoparticle-treated cells allowed interrogation of gene correction at the level of individual cells. Modification was passed on to cell progeny through months of cloning, demonstrating heritability. Gene modification in these positive clones was further confirmed by direct sequencing and deep sequencing. CFTR gene correction in the positive clones was also confirmed by the presence of sequence-corrected mRNA and by functional analysis in an MQAE chloride flux assay. Positive clones had increased the chloride flux in comparison with untreated F508del CFBE cells. Modified PLGA/PBAE/MPG nanoparticles loaded with the PNA and donor DNA showed improved activity over PLGA nanoparticles, as demonstrated by MQAE chloride flux and deep sequencing both in vitro and in vivo . Of note, PLGA/PBAE/MPG nanoparticles carrying PNA/DNA cargo targeting an unrelated genomic site did not produce changes in the chloride flux either in vitro or in vivo , suggesting that the observed effects are due to gene modification rather than a nonspecific physiologic effect. In other work, using nanoparticles loaded with fluorescent dyes as tracers, we demonstrated that intranasal administration of PLGA/PBAE/MPG nanoparticles produced significantly greater nanoparticle association with airway epithelial cells than PLGA nanoparticles [36] . After multiple in vitro treatments with PLGA/PBAE/MPG nanoparticles, the chloride efflux of CFBE cells approached that of normal HBE cells, and modification frequencies of up to 25% on the basis of functional chloride efflux. However, it is possible that some individual cells with increased efflux may have had enhanced chloride transport because of a bystander effect from being adjacent to corrected cells, and not from direct modification. In addition, it is possible that corrected cells have a selection advantage, resulting in their preferential expansion. Deep sequencing showed modification up to 10% and no off-target effects above background mutation/read error rates in untreated cells as assessed in 13 sites with partial homology for possible off-target binding of the PNA. In addition, no increased DNA damage was detected in treated cells using comet assay. This is expected, given that tail-clamp PNA molecules have very low levels of binding to mismatched sites and do not have any intrinsic nuclease activity. Unlike nuclease-based approaches to gene editing like ZFN and CRISPR, PNAs do not directly make strand breaks but instead provoke endogenous DNA repair pathways in the cell to mediate sequence conversion and gene correction that is templated by the co-introduced donor DNA. A low frequency of off-target effects will be of utmost importance for gene editing in this chronic, systemic disease. In addition, surface-modified PLGA/PBAE/MPG nanoparticles showed greater genome-engineering capacity after direct in vivo administration. Multiple intranasal treatments with PLGA/PBAE/MPG nanoparticles containing the murine CFTR -specific triplex-forming PNAs and donor DNAs were found to significantly modify the characteristic nasal potential difference defect in CF mice. Modification frequencies were greater than 5% in the nasal epithelium and 1% in the lung, with no detectable off-target mutations in a partially homologous site. There was no enhanced inflammatory cytokine production or changes in lung histology, highlighting the low immunogenicity of our approach. Because of this low toxicity, we speculate that longer courses of treatment are feasible and should enhance gene modification. Since correction of only one defective allele is required for restoration of the chloride flux in cells, and studies have indicated that as little as 6–10% of cells need to be corrected for normal levels of ion transport in culture [45] , our system has the potential to achieve gene correction at a clinically relevant level. While the work presented here provides a foundation for PNA-based gene editing of CFTR , there are still many avenues left unexplored for further improvement of this in vivo genome-engineering strategy. Future PNA designs to explore may include gamma-PNA molecules with a stereogenic mini-PEG group at the gamma position to enhance binding, use of guanidine-G-clamp PNA monomers to enhance PNA binding or PNA/peptide conjugates for increased nuclear PNA uptake. Improvements in nanoparticle formulation may include use of surface modifiers targeting specific cell types, exploration of new polymers developed by our laboratory and others for oligonucleotide delivery and formulation techniques to vary nanoparticle size. While we have shown that the combination of tail-clamp PNAs and PLGA/PBAE/MPG nanoparticles improves gene modification with triplex-forming oligonucleotides by an order of magnitude compared with previous approaches, there are still many possibilities for further enhancement of in vivo gene modification. In addition, for translation to clinical use, several avenues of study must be further explored, including inflammatory response in CF mouse animal models with more robust respiratory phenotypes [46] . Although the CF mouse model used in these studies has a mild respiratory phenotype that increases with age, the robust spontaneous pathology observed in the human disease process is not seen. One might consider using the ENaC-Tg-overexpressing mouse to model the ability of nanoparticles to penetrate thickened airway mucus; however, given that there is no underlying CFTR defect, the efficacy of gene-editing in such a model would be limited. In addition, the properties of CF mucus may be quite different from that of the ENaC-Tg model because of alterations in airway surface liquid pH and bicarbonate concentrations that have been reported in CF [47] , [48] . Alternatively, future studies could use house dust mite extracts to potentially induce mucus hyperproduction, which may better approximate the airway pathology observed in advanced CF lung disease. Other potential models to explore include the CF pig model [49] , which most closely mirrors human disease. Modification of lung epithelial progenitors would also be required for more long-term correction of the phenotype; while permanent genomic change using PNA/DNA is less transient than plasmid-based approaches and the changes will be passed on to daughter cells, some modified cells may be lost over time with regular turnover of the respiratory epithelium. In summary, we have shown that PNA/DNA-encapsulating nanoparticles can correct the F508del mutation in human CFBE cells, resulting in the appearance of CFTR-dependent chloride transport. We have also shown that intranasal treatment with PLGA/PBAE/MPG nanoparticles can correct the chloride flux as measured by changes in nasal potential difference measurements in a CF mouse model, and leads to gene modification in the lung. This is the first demonstration of the use of triplex-mediated recombination for gene correction in CFTR . Modified PLGA/PBAE/MPG nanoparticles showed enhanced efficacy over PLGA nanoparticles, allowing us to achieve site-specific gene modification at levels an order of magnitude higher than previously possible with the PNA technology. While ZFNs and CRISPR/Cas9 systems have previously been used for CFTR gene editing, gene modification has been at lower frequencies with higher off-target effects, and without a system for in vivo translation. The delivery vehicle presented here could be used for direct in vivo gene editing using other nucleic acid-based approaches, such as short fragment homologous recombination and CRISPR/Cas9 plasmid systems. Oligonucleotides PNAs with an 8-amino-2,6-dioxaoctanoic acid linker were purchased from Bio-Synthesis (Lewisville, TX) or Panagene (Daejeon, Korea) and purified using HPLC. Donor oligonucleotides 50 nt in length were synthesized by Midland Certified Reagent (Midland, TX), 5′- and 3′-end-protected by three phosphorothioate internucleoside linkages at each end and purified by reversed phase-HPLC. Sequences of PNA molecules used are given in Fig. 1 and Supplementary Fig. 1 . Human donor DNA sequence: 5′-TTCTGTATCTATATTCATCATAGGAAACACCAAAGATAATGTTCTCCTTAATGGTGCCAGG-3′ mouse donor DNA sequence: 5′-TCTTATATCTGTACTCATCATAGGAAACACCAAAGATAATGTTCTCCTTGATAGTACCCGG-3′. In our mismatched PNA control experiments, a PNA molecule targeting the human β-globin gene was used with 12 mismatches in the Watson Crick domain relative to the CF PNA2: JTTTJTTTJTJT-OOO-TCTCTTTCTTTCAGGGCA β-globin -targeted PNA TJTJJTTT-OOO-TTTCCTCTATGGGTAAGCFTR-targeted PNA. The β-globin -targeted PNA has 8 T, 5 C, 2 A, 3 G in the Watson–Crick domain and 8 T and 4 J in the Hoogsteen domain. The CFTR-targeted PNA has 7 T, 3 C, 3 A and 4 G in the Watson–Crick domain and 5 T and 3 J in the Hoogsteen domain. Gel shift assays for PNA binding To test the binding of candidate tail-clamp PNA molecules to the targeted site in the CFTR gene, PNA was incubated with plasmid DNA containing the target site at 37 °C overnight, with 10 μM KCl in TE at final volume of 10 μl. Samples were digested with restriction enzymes flanking the binding site (EcoRI and BamHI), and the products run on an 8% nondenaturing PAGE gel. A silver stain was used to visualize the products. Uncropped gel images are included in Supplementary Fig. 9 . Nanoparticle formulation and characterization PLGA nanoparticles loaded with PNA and DNA were formulated and characterized using a double-emulsion solvent evaporation technique as previously described [32] . Instead of 1:1 PNA:DNA, 1:2 PNA:DNA was loaded in each batch in initial screening studies (20 μl of 2 mM donor, 20 μl of 1 mM PNA per 80 mg of PLGA). For particles in subsequent studies, 80 nmol (40 μl of 2 mM solution) of PNA and 40 nmol (20 μl of 2 mM solution) of DNA were used per 80 mg particle batch (scaled up or down accordingly). Briefly, 80 mg of polymer was dissolved in 160 μl dichloromethane overnight. PNA and DNA were dissolved in RNase/DNase-free water. The PNA and DNA were then added dropwise into the dissolved polymer while vortexing, and then sonicated for 10 s three times (Tekmar Probe Sonicator, Cincinatti, OH). The polymer solution was then added dropwise to 3.2 ml of 5% poly (vinyl alcohol) (PVA) while vortexing, and then sonicated for 10 s three times using a probe sonicator on ice. The emulsion was then transferred to 20 ml of 0.3% PVA in a beaker with a stir bar, and left for 3 h to let the solvent evaporate. This solution was then washed three times using ultracentrifugation with 10 ml of water, and then resuspended in 2.5 ml of water and transferred into Eppendorf tubes. Eppendorfs were frozen at −80 °C for at least 2 h, and then transferred to a lyophilizer for 3 days. PBAE was synthesized by a Michael addition reaction of 1,4-butanediol diacrylate (Alfa Aesar Organics, Ward Hill, MA) and 4,4′-trimethylenedipiperidine (Sigma, Milwaukee, WI) as previously reported [50] . DSPE-PEG(2000)-maleimide was purchased from Avanti Polar Lipids (Alabaster, AL). MPG peptides were purchased from Keck (Yale University). Cell penetrating peptides (CPPs) were covalently linked to DSPE-PEG-maleimide as previously reported [35] . PLGA/PBAE particles contained 15% PBAE (wt%), and solvent from these particles was evaporated overnight in PVA instead of for 3 h as above. To make surface-modified particles, DSPE-PEG-MPG was added to the 5.0% PVA solution during formation of the second emulsion at a 5 nmol mg −g ligand-to-polymer ratio. In subsequent studies, particles were loaded as indicated. SEM imaging and controlled release studies were performed as before [32] . Briefly, for SEM imaging, particles were sputter-coated with gold before imaging. For controlled release studies, particles were dissolved in 600 μl of DNase/RNase-free water, put in a 37 °C shaker and at set time points centrifuged at 13,000 r.p.m. in a microfuge; at each time point, the supernatant was examined using a NanoDrop 8000 for nucleic acid content. Cell culture CFBE cells (CFBE41o-) and HBE cells (16HBE14o-) [38] were grown with LHC-8 media (Invitrogen) with 10% fetal bovine serum, 1 × antibiotic antimycotic (Gibco) and tobramycin 40 mg per 500 ml (Sigma). Once grown to confluence, cells were trypsinized by first washing with 0.05% trypsin, then adding 0.25% trypsin for 5 min and then harvesting with RPMI medium with 10% fetal bovine serum. Cells were frozen in 5% dimethylsulphoxide in culture medium as necessary. Nanoparticles were resuspended in culture media by vigorous vortexing and water sonication, and then added directly to cells at concentrations of 2 mg ml −1 per 1 × 10 6 cells (corresponding to ∼ 10 9 PNA/DNA molecules delivered to each cell assuming 100% efficiency). To test primers, a 712-base pair region of the CFTR gene, with either the F508DEL or corrected sequence (including our silent modifications), was cloned into plasmids. PCR reactions were first tested on plasmids. Gradient and step-down PCR at varying conditions was performed to ensure that F508del primers only amplified the F508del plasmid, and the donor-specific primers only amplified the donor-sequence-containing plasmids. Primers are included in Supplementary Table 2 . Genomic DNA extraction and AS-PCR Genomic DNA was harvested from cells and purified using the Wizard Genomic DNA Purification kit (Promega, Madison, WI). Equal amounts of genomic DNA from each sample were subjected to allele-specific PCR, with a gene-specific reverse primer, and an allele-specific forward primer in which the 3′ end corresponds to the 6-bp-modified sequence. Quantitative PCR was performed using a Stratagene Mx 3000 P cycler. Donor DNA (0.2 μM) was used in spiking experiments. Copy numbers of DNA in the PCR reaction were ∼ 10 14 copies of genomic DNA and 10 12 copies of spiked donor DNA. PCR products were separated on a 1% agarose gel and visualized using a gel imager. Relative gene modification was calculated using the 2 −ΔΔ C t method, with the average of the untreated controls used as the reference groups [51] . AS-PCR conditions are as follows. Platinum Taq polymerase (Invitrogen, Carlsbad, CA) was used for PCR reactions: 5 μl betaine, 4.25 μl water, 2.5 μl 10 × Platinum Taq PCR buffer, 1.25 μl 50 mM MgCl 2 , 0.5 μl dNTPs, 0.5 μl each primer at 10 μM, 0.5 μl Platinum Taq polymerase and 10 μl of genomic DNA at 40 ng μl −g . PCR cycler conditions for human CFTR were as follows: 95 °C 2 min, 94 °C 30 s, 69 °C 1 min, 72 °C 1 min, 94 °C 30 s, 68 °C 1 min, 72 °C 1 min, 94 °C 30 s, 67 °C 1 min, 72 °C 1 min, 94 °C 30 s, 66 °C 1 min, 72 °C 1 min, 94 °C 30 s, 65 °C 1 min, 72 °C 1 min, (94 °C 30 s, 65 °C 1 min, 72 °C 1 min) × 35 cycles, 72 °C 2 min, hold at 4 °C 1. PCR cycler conditions for mouse CFTR were as follows: 94 °C for 5 min (94 °C 30 s, 66.9 °C (for detection of F508del) or 68.3 °C (for detection of modification) 45 s, 72 °C 1 min) × 40, 72 °C 6 min, hold at 4 °C. Conditions were optimized using plasmids containing the target sequences as indicated above. Of note, our donor sequences contain an additional four base pairs of silent mutations distinguishing the donor sequence from wild-type CFTR , to ensure that contaminating wild-type cells (environmental or from other cell cultures) do not appear as false-positives. Uncropped gel image is included in Supplementary Fig. 10 . For regular sequencing, High Fidelity Platinum Taq Polymerase (Invitrogen) was used. PCR conditions for production of amplicons for regular sequencing were as follows: 0.5 μl dNTPs, 2.5 μl 10 × HiFi Buffer, 1.5 μl 50 mM MgCl 2 , 14.1 μl water, 0.4 μl Taq HiFi, 0.5 μl each primer at 10 μM, 5 μl genomic DNA at 80 ng μl −g . PCR cycler conditions were as follows: 94 °C 2 min (94 °C 30 s, 55 °C 45 s, 68 °C 1 min) × 35, 68 °C 1 min, hold at 4 °C. RNA extraction and reverse-transcription AS-PCR The RNAeasy Plus Qiagen Kit (Gaithersburg, MD) was used to extract RNA, and the Invitrogen superscript III kit (Carlsbody, CA) was used to make cDNA. PCR reactions contained cDNA, 20% Betaine, 0.2 mM dNTPs, Advantage 2 Polymerase Mix, 0.2 μM of each primer and 2% platinum taq. Gene-specific reverse primer: 5′-CCTAGTTTTGTTAGCCATCAGTTTACAGAC-3′, F508DEL CF primer: 5′-GCCTGGCACCATTAAAGAAAATATCATTGG-3,′ primer for corrected/donor: 5′-CCTGGCACCATTAA G GA G AA C AT T AT CTT -3′. PCR cycler conditions were as follows: 95 °C 5 min (95 °C 30 s, 65 °C 1 min, 72 °C 1 min) × 35, 72 °C 5 min, hold at 4 °C. Deep sequencing Genomic DNA was isolated from treated cells or mouse tissue, and PCR reactions performed with high-fidelity TAQ polymerase. Each PCR tube consisted of 28.2 μl dH 2 O, 5 μl 10 × HiFi Buffer, 3 μl 50 mM MgCl 2 , 1 μl DNTP, 1 μl each of forward and reverse primer, 0.8 μl HiFi Platinum Taq and 10 μl DNA template. Separate barcoded primers (6 bp barcode plus primer) were used for each sample. PCR conditions were as follows: for regular sequencing, High Fidelity Platinum Taq Polymerase (Invitrogen) was used. PCR conditions for production of amplicons for regular sequencing were as follows: 0.5 μl dNTPs, 2.5 μl 10 × HiFi Buffer, 1.5 μl 50 mM MgCl 2 , 14.1 μl water, 0.4 μl Taq HiFi, 0.5 μl each primer at 10 μM, 5 μl genomic DNA at 80 ng μl −1 . PCR cycler conditions were as follows: 94 °C 2 min (94 °C 30 s, 55 °C 45 s, 68 °C 1 min) × 35, 68 °C 1 min, hold at 4 °C. PCR products were prepared by end-repair and adapter ligation according to the Illumina protocols (San Diego, CA), and pooled samples were sequenced by the Illumina HiSeq with 75 paired-end reads at the W.M. Keck Facility at Yale University. Sequences have been uploaded to http://www.ncbi.nlm.nih.gov/bioproject/276283 . Analysis was performed using a software designed by Nicole McNeer and Ken Hui (Yale School of Medicine), PERL file available as Supplementary Software online, and using software designed by Yong Kong (associate director Yale Bioinformatics Resource Center), code available at http://graphics.med.yale.edu/trim/ . The programme Btrim was used to trim off low-quality regions of each read and to assign the trimmed reads to each barcode [52] . The number of reads with modified sequence or original sequence were also searched by using Btrim. For off-target sites, the trimmed reads were mapped using programme bowtie2 (ref. 53 ). Primers are listed in Supplementary Table 2 . MQAE assay for chloride flux MQAE is a chloride-sensitive fluorescent dye we used to assess the chloride flux in plated CFBE cells as previously described [40] . Cells were grown to confluence directly on coverslips. Then, cells were placed in Cl-containing solution (135 mM NaCl, 5 mM KCl, 1 mM CaCl 2 , 1.2 mM MgSO 4 , 2 mM NaH 2 PO 4 , 2 mM HEPES and 10 mM glucose), and then moved to a chloride-free solution (135 mM NaCyclamate, 3 mM KGluconate, 0.5 mM CaCyclamate, 1.2 mM MgSO 4 , 2 mM KH 2 PO 4 , 2 mM HEPES and 10 mM glucose). Finally, the chloride flux was assessed in solution with forskolin (10 μM) and IBMX (100 μM) was added. MQAE experiments were performed on an Olympus IX-71 inverted microscope, with MQAE excited at 354 nm and fluorescence measured at 460 nm every 5 s. Fluorescence was measured on a cell-by-cell basis, with 30–100 cells catalogued per slide. The rate of change in MQAE fluorescence (arbitrary fluorescence units (AFU) per time) was graphed, and AFU per min was compared between groups. Graphs shown are normalized to background. Animal model We used a mouse model homozygous for the F508del mutation on a fully backcrossed C57/BL6 background [42] . Mice were between 12 and 40 weeks of age (the majority between 3 and 6 months of age), an equal mix of male and female. Nanoparticles were resuspended at 1 mg in 50 μl PBS, sonicated and administered to mice by intranasal instillation. Mice were treated with a total of 7 mg of nanoparticles over a course of 2 weeks (one treatment every other day)—this corresponds to a total of ∼ 3.5 nmoles of donor DNA ( ∼ 10 15 copies) and 7 nmol of PNA per mouse ( ∼ 2 × 10 15 copies). Estimating ∼ 400 million cells per mouse lung, this corresponds to ∼ 5 million PNA and 2.5 million DNA molecules per murine lung cell, if delivery to the lung is 100% efficient. Control mice were treated identically with either blank nanoparticles without nucleic acid cargo or with nanoparticles containing PNA/DNA targeting human β-globin . While a scrambled PNA would provide the most closely matched molecular control, this off-target PNA provides a control of effects from nonspecific PNA activity. Each independently performed experiment included at least one CF-targeted PNA/DNA-treated mouse and one control mouse. All procedures were performed in compliance with relevant laws and institutional guidelines, and were approved by the Yale University Institutional Animal Care and Use Committee. NPDs were measured as previously described [5] . Briefly, mice were anaesthetized with ketamine/xylazine, and one electrode probe placed into one nostril, with a reference electrode with 3% agar in Ringer’s solution placed subcutaneously. A microperfusion pump was used to flow the solution through the electrode probe at 0.2 ml h −1 . Potential differences were measured first with a control Ringer’s solution, then with Ringer’s solution containing 100 μM amiloride, then a chloride-free solution with amiloride and then chloride-free solution with amiloride and forskolin/IBMX. NPDs were measured before and after the nanoparticle treatment. BAL fluid analysis and lung histology BAL fluid was collected by standard protocols as previously described [54] , and cytokines measured using a microsphere-based multiplex assay as per the manufacturer’s instructions (Luminex; Millipore, Billerica, MA). To collect the lungs for histopathology, a midline incision from the sternum to the diaphragm was made and, to remove blood from the pulmonary circulation, PBS was perfused via the right ventricle using a 20-g needle. Lungs were inflated with 0.5% low melt agarose at constant pressure, and then removed from the chest and placed in fixative. Paraffin-embedded tissues were stained with haemotoxylin and eosin stain for imaging. Comet assay Overall, 300,000 CFBE cells per well were plated on six-well plates in 1 ml media, and then treated with 2 mg ml −1 of PBAE/MPG/PLGA nanoparticles either with DNA alone or with both DNA and PNA, or with lipofectamine to deliver 2 μg of human cas9 plasmid no. 41815 (Addgene, Cambridge, MA) [43] . After 24 h, cells were scraped and harvested, and prepared using the Trevigen CometAssay kit as per the manufacturer’s protocol (Trevigen, Gaithersburg, MD). Briefly, cells were suspended in agarose, added to comet slides, allowed to set, incubated for 1 h in lysis solution, placed in electrophoresis solution for 30 min, then run at 21 V for 45 min, placed in acetate solution for 30 min, 70% ethanol solution for 30 min, dried, stained with Sybr Green for 30 min and then visualized using an EVOS microscope. TriTek Comet Score freeware was used to analyse the images. Data analysis Data are represented as individual data points or as mean and s.e.m. unless otherwise indicated. Data analysis was performed with the Excel and Prism commercial software. Statistical significance was determined using Student’s t -test, two-tailed, unpaired or Fisher’s exact test. The code used for deep-sequencing analysis is available at http://graphics.med.yale.edu/trim/ . Accession codes. The sequences generated by deep sequencing have been deposited in SRA database under the accession codes (awaiting upload). Sequences have been uploaded to http://www.ncbi.nlm.nih.gov/bioproject/276283 . How to cite this article: McNeer, N. A. et al. Nanoparticles that deliver triplex-forming peptide nucleic acid molecules correct F508del CFTR in airway epithelium. Nat. Commun. 6:6952 doi: 10.1038/ncomms7952 (2015).